Bats host major mammalian paramyxoviruses The large virus family Paramyxoviridae includes some of the most significant human and livestock viruses, such as measles-, distemper-, mumps-, parainfluenza-, Newcastle disease-, respiratory syncytial virus and metapneumoviruses. Here we identify an estimated 66 new paramyxoviruses in a worldwide sample of 119 bat and rodent species (9,278 individuals). Major discoveries include evidence of an origin of Hendra- and Nipah virus in Africa, identification of a bat virus conspecific with the human mumps virus, detection of close relatives of respiratory syncytial virus, mouse pneumonia- and canine distemper virus in bats, as well as direct evidence of Sendai virus in rodents. Phylogenetic reconstruction of host associations suggests a predominance of host switches from bats to other mammals and birds. Hypothesis tests in a maximum likelihood framework permit the phylogenetic placement of bats as tentative hosts at ancestral nodes to both the major Paramyxoviridae subfamilies ( Paramyxovirinae and Pneumovirinae ). Future attempts to predict the emergence of novel paramyxoviruses in humans and livestock will have to rely fundamentally on these data. The ability to predict and prevent viral epidemics has become a major objective in the public health disciplines. Knowledge of viral hosts enables the identification of maintenance populations from which epidemics may emerge [1] , [2] , [3] , [4] . From an ecological perspective, the natural host of a given virus may be regarded as its habitat [5] , [6] . Unfortunately, unbiased assessment of habitat is impossible, as it requires the investigation of all host species in all possible geographical locations. Moreover, the delimitations of viral species and populations are often not well defined. However, viral phylogenies can identify whether extant viruses encountered in a given host are less or more directly linked to common ancestors, providing clues to virus origins [4] , [5] , [6] . Hosts of relevant infectious disease agents share distinctive properties that can be summarised into a cumulative definition of animal reservoirs (AR) as of interest in public health. We define as ARs those taxa of extant animals that contain higher genetic virus diversity than target taxa, harbour the virus continuously on the level of social groups (with or without disease) [4] , [7] , and are naturally infected beyond the geographical limits of communicating social groups [3] , [4] . These cumulative parameters are amenable to field investigations, without the requirement to manipulate wild animals and their habitats extensively. Nevertheless, logistical, ethical and ecological limits in field investigations still require a focussing on appropriate candidate taxa. Here, it is helpful to consider that the potential of animals to act as AR can be linked to social and behavioural parameters, which in turn are inherent to taxa. Virus transmission and maintenance is generally favoured by large social groups, close social interaction, high population densities, as well as spatial mobility and fast population turnover [2] , [4] , [8] . It is also helpful to consider that genetic proximity between species is favourable of cross-species pathogen transmission [6] , [9] , [10] , [11] . For instance, all cumulative criteria are met by the best studied of relationships between a virus genus and its AR, the influenza A virus in waterfowl [3] , [9] , [10] . In applying the above considerations to larger taxa of mammalian viruses, such as the members of the mammalian paramyxoviruses (PVs), mammals come into focus as potential AR. In mammals, the criterion of large natural group sizes is particularly met by species within the orders Chiroptera (bats) and Rodentia (rodents) [1] , [8] . Indeed, sporadic detection of PV in members of both orders has been previously reported by us and other groups [12] , [13] , [14] , [15] , [16] . Here we tested 119 bat and rodent species worldwide, and identified a large range of novel PV related to major pathogens. These included very large diversities of henipa- and rubulaviruses, as well as relatives of respiratory syncytial virus (RSV), mouse pneumonia- and canine distemper virus in bats. Multiple morbilli-related viruses were found in bats and rodents. These data will change our conception of PV host associations and influence future attempts to assess and predict epidemic risks. PV detection in small mammals To assess the spectrum of PV in bats and rodents, 86 species of bats (4,954 individuals) and 33 species of rodents (4,324 individuals) were sampled in 15 locations worldwide ( Fig. 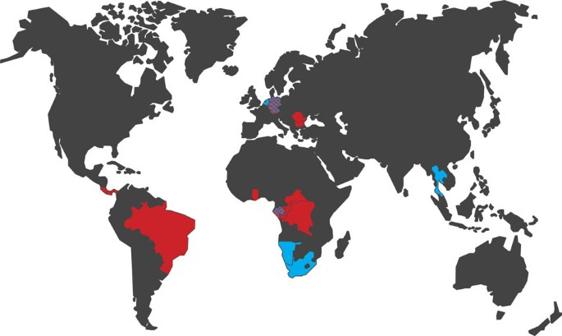Figure 1: Sampling sites and specimens. The bat samples used in this study and their countries of origin are depicted in red, rodent samples in blue. Sampled animals are listed by species inTable 1. Numbers indicate paramyxovirus-positive individuals and individuals tested in total. DRC=Democratic Republic of Congo, RCA=Central African Republic. Sampling years and results of individual RT–PCR assays are given inSupplementary Table S1. 1 , Table 1 and Supplementary Table S1 ). All samples were screened for Paramyxoviridae by various reverse transcription (RT)–PCR assays. Pooled serum samples were additionally screened by random amplification and deep sequencing of serum-derived cDNA. Although this approach identified a range of viruses whose full genomes remain to be determined, no PVs were detected ( Supplementary Table S2 ). This was presumably due to higher concentrations of the identified viruses in blood, or because of properties that technically promote detection by random amplification, such as circularity of DNA genomes. In contrast, RT–PCR detected a large range of PV cDNA sequences as described below. Figure 1: Sampling sites and specimens. The bat samples used in this study and their countries of origin are depicted in red, rodent samples in blue. Sampled animals are listed by species in Table 1 . Numbers indicate paramyxovirus-positive individuals and individuals tested in total. DRC=Democratic Republic of Congo, RCA=Central African Republic. Sampling years and results of individual RT–PCR assays are given in Supplementary Table S1 . Full size image Table 1 Full size table Phylogenies were inferred using maximum likelihood and Bayesian approaches ( Fig. 2a–e and Supplementary Fig. S1 ). Detection rates of viruses in bats and rodents were similar at 3.3 and 3.1%, respectively, but bat viruses were dispersed across the phylogenetic tree with pronounced genetic divergence, whereas rodent viruses belonged to three clades with relatively low divergence that were not exclusively detected in rodents ( Supplementary Fig. S1 ). PVs were detected in six of ten families of bats tested, representing all major chiropteran phylogenetic lineages ( Fig. 3a,b ). A simplified criterion based on pairwise amino acid distance matrices was used to estimate how many novel virus species might have been detected (refer to Methods section). In total, 66 novel PV taxa at the level of putative species were discernible. This number exceeded the number of PV species currently known, as the International Committee on Taxonomy of Viruses (ICTV) currently lists 36 species, and even upon inclusion of unclassified sequences from GenBank, only an estimated 57 species can be discerned. 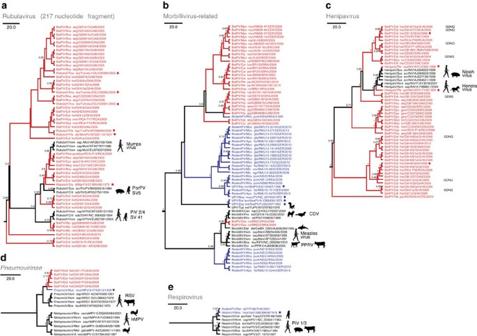Figure 2: PartialL-gene phylogenies including novel paramyxoviruses (PVs) from small mammals. The generaRubulavirus(a),Morbillivirus(b),Henipavirus(c) andRespirovirus(e), as well as the subfamilyPneumovirinae(d) are shown with bat viruses coloured in red and rodent viruses in blue. Major PVs are indicated by a pictogram of typical ordinal host and designations of virus species (SV, simian virus; PorPV, porcine PV; PIV, parainfluenzavirus; CDV, canine distemper virus; PPRV, peste des petits ruminants virus; RSV, respiratory syncytial virus; hMPV, human metapneumovirus). Bat and rodent viruses marked by an asterisk have been described previously. Values at node points indicate Bayesian posterior probabilities of grouping (only values above 0.6 are shown). The scale bar indicates substitutions per site. For selected henipaviruses (c), the four amino acid GDNE/GDNQ motif at the catalytic site of the RNA-dependent RNA polymerase is shown. Abbreviations used in virus designations are detailed inSupplementary Table S1. Figure 2: Partial L -gene phylogenies including novel paramyxoviruses (PVs) from small mammals. The genera Rubulavirus ( a ), Morbillivirus ( b ), Henipavirus ( c ) and Respirovirus ( e ), as well as the subfamily Pneumovirinae ( d ) are shown with bat viruses coloured in red and rodent viruses in blue. Major PVs are indicated by a pictogram of typical ordinal host and designations of virus species (SV, simian virus; PorPV, porcine PV; PIV, parainfluenzavirus; CDV, canine distemper virus; PPRV, peste des petits ruminants virus; RSV, respiratory syncytial virus; hMPV, human metapneumovirus). Bat and rodent viruses marked by an asterisk have been described previously. Values at node points indicate Bayesian posterior probabilities of grouping (only values above 0.6 are shown). The scale bar indicates substitutions per site. For selected henipaviruses ( c ), the four amino acid GDNE/GDNQ motif at the catalytic site of the RNA-dependent RNA polymerase is shown. Abbreviations used in virus designations are detailed in Supplementary Table S1 . 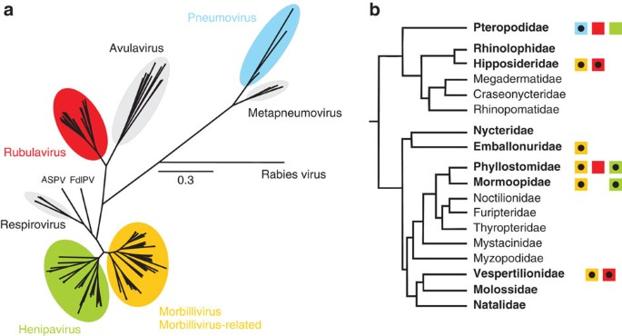Figure 3: Bat paramyxovirus (PV) dispersion among bat host families. (a) Maximum likelihood phylogeny reconstructed from 186 amino acids of theL-gene corresponding to positions 367–552 in NiV strain UM-0128 RNA-dependent RNA polymerase (GenBank, AJ564623) withParamyxoviridaegenera shown in blue, red, green and yellow colour. Rabies virus, Atlantic salmon PV (ASPV), Fer-de-lance PV (FdlPV) and genera not containing bat viruses are shaded in grey. The scale bar represents evolutionary distance in substitutions per site. (b) Chiropteran phylogeny adapted from Simmons60. Those bat families sampled in this study are shown in bold type. Detected PV genera per bat family are symbolised by squares coloured as in (a). Black dots in rectangles indicate virus-host pairs (bat families versus bat genera) identified for the first time in this study. The approximate numbers of bat species per family were as follows: Vespertilionidae (more than 350), Pteropodidae (about 200), Phyllostomidae (about 190), Molossidae (about 100), Hipposideridae (about 90, including Rhinopomatidae), Rhinolophidae (about 80), Emballonuridae (about 50), Megadermatidae (about 5), Nycteridae (about 20), Natalidae (about 5), Thyropteridae (about 5), Noctilionidae (2), Myzopodidae (2), Mystacinidae (1), Furipteridae (1). Full size image Figure 3: Bat paramyxovirus (PV) dispersion among bat host families. ( a ) Maximum likelihood phylogeny reconstructed from 186 amino acids of the L -gene corresponding to positions 367–552 in NiV strain UM-0128 RNA-dependent RNA polymerase (GenBank, AJ564623) with Paramyxoviridae genera shown in blue, red, green and yellow colour. Rabies virus, Atlantic salmon PV (ASPV), Fer-de-lance PV (FdlPV) and genera not containing bat viruses are shaded in grey. The scale bar represents evolutionary distance in substitutions per site. ( b ) Chiropteran phylogeny adapted from Simmons [60] . Those bat families sampled in this study are shown in bold type. Detected PV genera per bat family are symbolised by squares coloured as in ( a ). Black dots in rectangles indicate virus-host pairs (bat families versus bat genera) identified for the first time in this study. The approximate numbers of bat species per family were as follows: Vespertilionidae (more than 350), Pteropodidae (about 200), Phyllostomidae (about 190), Molossidae (about 100), Hipposideridae (about 90, including Rhinopomatidae), Rhinolophidae (about 80), Emballonuridae (about 50), Megadermatidae (about 5), Nycteridae (about 20), Natalidae (about 5), Thyropteridae (about 5), Noctilionidae (2), Myzopodidae (2), Mystacinidae (1), Furipteridae (1). Full size image Major PV genera in bats The genus Rubulavirus contains three human pathogens, the mumps virus, as well as the respiratory viruses, Parainfluenzavirus 2 and 4 . A large range of novel rubulaviruses in fruit- and insect-eating African bats were identified in addition to those six bat rubulaviruses previously known ( Fig. 2a , Supplementary Table S1 ). The viruses could be classified into 21 discernible taxonomic entities on the level of putative species. No rubulaviruses were detected in rodents. A bat virus of high similarity to mumps virus was fully sequenced from a bat spleen (15,378 nucleotides, ( Supplementary Fig. S2 )). Amino acid similarity was well above 90% in all genes except P (89.5%), suggesting this virus and human mumps to be conspecific. To determine antigenic relatedness to human mumps virus, sera from 52 flying foxes and 78 insect-eating bats were tested by immunofluorescence ( n =26 Eidolon helvum , 5 Epomops franqueti , 5 Micropterus pusillus , 5 Myonycteris torquata , 11 Rousettus aegyptiacus , 14 Coleura afra , 21 Hipposideros cf. caffer , 11 Hipposideros gigas , 17 Miniopterus inflatus , 11 Rhinolophus cf. alcyone ). Clear reactivity was observed in 41.5% of the 130 tested bat sera ( Fig. 4a ). Specificity of these reactivities was confirmed by cross-testing against other PVs, including the rubulavirus Parainfluenzavirus 2 ( Fig. 4b ). These data in total suggest that mumps and related bat viruses may belong to one same serogroup. 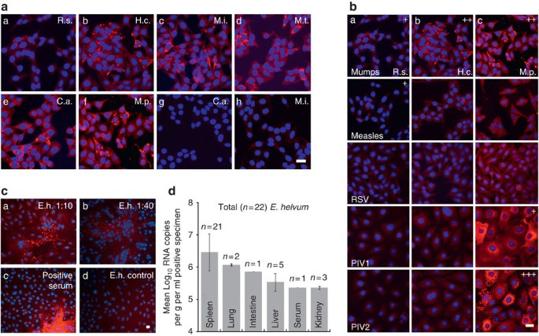Figure 4: Serology and virus concentrations for selected bat PV. (a) Reactivity of different sera (diluted 1/40) from African bats with human mumps virus in Vero cells by indirect immunofluorescence assay, a) Rhinolophidae (R.s.,Rhinolophus sp.), b) Hipposideridae (H.c.,Hipposideros ruber/caffer), c) Vespertilionidae (M.i.,Miniopterus inflatus), d) Pteropodidae (M.t.,Myonycteris torquata), e) Emballonuridae (C.a.,Coleura afra), f) Pteropodidae (M.p.,Micropteropus pusillus), g) and h) non-reactive sera from C.a and M.i. (b) Prototype PVs mumps, measles, RSV, parainfluenza 1 (PIV1) and PIV2 infected in Vero cells, stained with bat sera R.s., H.c., M.p. as above. Signal intensities were rated from negative to +++. (c) Reactivity ofEidolon helvum(E.h., sample GH64) serum from Ghana with NiV antigen using an indirect immunofluorescence assay: a) and b) represent 1/10 and 1/40 dilution of E.h. serum, c) positive control using a guinea pig anti-NiV serum, including a large NiV-induced syncytia stained in red, and d) E.h. serum GH64 diluted 1/10 applied on non-infected cells. Bars in a, b and c represent 50 μm. All panels used the same microscope and camera settings to demonstrate the strength of cross-reactivity between NiV and African viruses. (d) Henipavirus RNA concentrations in 22E. helvumsolid organs and serum, of which 21 tested positive in spleens, 5 in livers, 3 in kidneys, 2 in lungs, 1 in intestine and 1 in serum. Virus concentrations (log10RNA copies per millilitre of serum or per gram of tissue) are given on theyaxis for each bat organ tested. Organ types are identified on thexaxis. Bars represent mean virus concentrations per organ type, whiskers show s.d. Figure 4: Serology and virus concentrations for selected bat PV. ( a ) Reactivity of different sera (diluted 1/40) from African bats with human mumps virus in Vero cells by indirect immunofluorescence assay, a) Rhinolophidae (R.s., Rhinolophus sp . ), b) Hipposideridae (H.c., Hipposideros ruber/caffer ), c) Vespertilionidae (M.i., Miniopterus inflatus ), d) Pteropodidae (M.t., Myonycteris torquata ), e) Emballonuridae (C.a., Coleura afra ), f) Pteropodidae (M.p., Micropteropus pusillus ), g) and h) non-reactive sera from C.a and M.i. ( b ) Prototype PVs mumps, measles, RSV, parainfluenza 1 (PIV1) and PIV2 infected in Vero cells, stained with bat sera R.s., H.c., M.p. as above. Signal intensities were rated from negative to +++. ( c ) Reactivity of Eidolon helvum (E.h., sample GH64) serum from Ghana with NiV antigen using an indirect immunofluorescence assay: a) and b) represent 1/10 and 1/40 dilution of E.h. serum, c) positive control using a guinea pig anti-NiV serum, including a large NiV-induced syncytia stained in red, and d) E.h. serum GH64 diluted 1/10 applied on non-infected cells. Bars in a, b and c represent 50 μm. All panels used the same microscope and camera settings to demonstrate the strength of cross-reactivity between NiV and African viruses. ( d ) Henipavirus RNA concentrations in 22 E. helvum solid organs and serum, of which 21 tested positive in spleens, 5 in livers, 3 in kidneys, 2 in lungs, 1 in intestine and 1 in serum. Virus concentrations (log 10 RNA copies per millilitre of serum or per gram of tissue) are given on the y axis for each bat organ tested. Organ types are identified on the x axis. Bars represent mean virus concentrations per organ type, whiskers show s.d. Full size image Measles is one of the most important childhood diseases. Measles virus defines the genus Morbillivirus that also contains the canine and phocine distemper virus, a dolphin morbillivirus, as well as Rinderpest and Peste Des Petits Ruminants viruses. Novel members of the genus Morbillivirus as currently defined by the ICTV were detected for the first time in bats (neotropical vampire bats) but not in rodents ( Fig. 2b ). A clade of morbillivirus-related rodent- and tupaia viruses, forming an unclassified sister clade to the genus Morbillivirus , was extended by an estimated 25 novel bat and rodent viruses, confirming the unclassified genus and the Morbillivirus genus to form a major stem lineage of PV. The genus Henipavirus comprises two known virus species causing fatal encephalitis in humans. These viruses (Hendra virus (HeV) in Australia, Nipah virus (NiV) in Asia) have been sporadically acquired from bats of the Pteropus genus by humans, swine and horses. We have recently detected small sequence fragments of potentially related viruses in a colony of E. helvum fruit bats in Ghana [12] . The present data identify at least 23 distinct viral clades in phylogenetic relation to henipaviruses in six bat species sampled in five different African countries ( Fig. 2c ). On the basis of the minimal genetic distance between HeV and NiV (7% in the analysed L -gene fragment), the African viruses were estimated to pertain to 19 novel virus species in the genus Henipavirus ( Figs 2c and 5 ). Full genome sequencing of a representative virus (GH-M74a) from a bat spleen confirmed formal classification in the genus Henipavirus (18,530 nucleotides, ( Supplementary Fig. S3 )). It was noted that the RdRp gene of the analysed African virus contained the catalytic motif GDNQ, as typical of the order Mononegavirales , whereas HeV and NiV have an atypical GDNE motif. Sequencing of this motif in representatives of all major African virus clades also yielded GDNQ, supporting the idea that African rather than Asian viruses are identical to generic ancestors in this highly conserved motif. In addition, the GDNE signature typical of HeV and NiV was found in a small fraction of African viruses, and these were in closest phylogenetic relationship to HeV and NiV ( Fig. 2c ). The most parsimonious explanation for the diversion of signatures in this highly conserved motif was a single change in a common ancestor to the GDNE-containing clade, as opposed to hypothetical convergent acquisitions of GDNQ in all but one of the parallel lineages. The GDNE-ancestral virus would most likely have existed in Africa, and would have been ancestral to HeV and NiV as well. 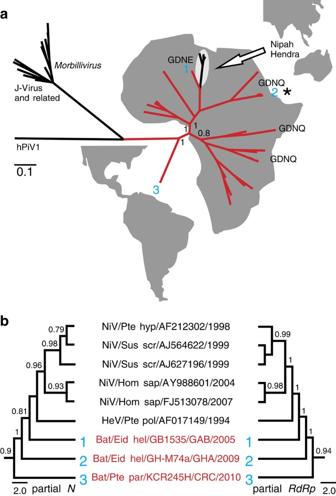Figure 5: Phylogeny of henipaviruses. (a) Bayesian phylogeny (WAG model) of the genusHenipavirusand sister generaMorbillivirusandJeilong(J-virus) showing novel bat viruses in red colour. Human parainfluenzavirus 1 (hPIV1) was used as an outgroup. Blue numbers represent viruses also represented in (b). The asterisk indicates the virus from which the full genomic sequence was analysed. For selected henipavirus clades, the four amino acid GDNE/GDNQ motif at the catalytic site of theRNA-dependant RNA polymeraseis shown. The scale shows amino acid substitutions per site in a translated 558 ntL-gene fragment, corresponding to positions 367–557 in NiV strain UM-0128L-gene (GenBank, AJ564623). (b) Bayesian nt-based phylogenies (GTR+G+I model) using a 642 ntN-gene fragment (left) corresponding to positions 401–1,042 in NiV strain UM-0128 and the 558 ntL-gene fragment (right). GB1535, virus fromEidolon helvum, Gabon; M74a,E. helvum(full genome available), Ghana; KCR245H,Pteronotus parnellii, Costa Rica. Numbers at nodes indicate Bayesian posterior probabilities. The scale bar represents nt substitutions per site. Figure 5: Phylogeny of henipaviruses. ( a ) Bayesian phylogeny (WAG model) of the genus Henipavirus and sister genera Morbillivirus and Jeilong (J-virus) showing novel bat viruses in red colour. Human parainfluenzavirus 1 (hPIV1) was used as an outgroup. Blue numbers represent viruses also represented in ( b ). The asterisk indicates the virus from which the full genomic sequence was analysed. For selected henipavirus clades, the four amino acid GDNE/GDNQ motif at the catalytic site of the RNA-dependant RNA polymerase is shown. The scale shows amino acid substitutions per site in a translated 558 nt L -gene fragment, corresponding to positions 367–557 in NiV strain UM-0128L-gene (GenBank, AJ564623). ( b ) Bayesian nt-based phylogenies (GTR+G+I model) using a 642 nt N -gene fragment (left) corresponding to positions 401–1,042 in NiV strain UM-0128 and the 558 nt L -gene fragment (right). GB1535, virus from Eidolon helvum , Gabon; M74a, E. helvum (full genome available), Ghana; KCR245H, Pteronotus parnellii , Costa Rica. Numbers at nodes indicate Bayesian posterior probabilities. The scale bar represents nt substitutions per site. Full size image Close relatedness between NiV and these African viruses was also demonstrated by immunofluorescence staining. To this end, Vero cells were infected in a biosafety level 4 laboratory with NiV and incubated with serum from E. helvum before staining with a polyclonal anti-bat antibody. Clear reactivity was seen ( Fig. 4c ). In two different widely distributed species of New World bats, one frugivorous ( Carollia perspicillata , rate 0.5%) and one insectivorous ( Pteronotus parnellii , rate 7.5%), we identified virus sequences that were phylogenetically closely related to the genus Henipavirus (area of distribution shown in Supplementary Fig. S4 ). These viruses formed a sister clade to the genus Henipavirus , including its novel African representatives ( Figs 2c and 5a ). It was impossible for ethical and logistical reasons to euthanise Neotropical bats and sample internal organs that might have enabled the completion of full genome sequences. Nevertheless, the N protein gene at the far opposite end of the genome of one of these viruses was successfully sequenced from a faecal sample. RdRp - and N -gene fragments were phylogenetically congruent and no signs of genomic recombination were seen ( Fig. 5b ). RSV and the related human metapneumovirus, belonging to the Pneumovirinae subfamily, are the leading causes of morbidity and mortality in children worldwide. We identified a clade of novel bat viruses also in this subfamily, which formed a sister clade to the human and bovine RSV ( Fig. 2d ). No bat viruses were detected in direct relationship to the genus Metapneumovirus , whose only human member, the human metapneumovirus, is most closely related to avian metapneumovirus C. These data support the notion that the metapneumoviruses are of direct avian, rather than direct mammalian descent [17] . Sendai virus, a member of the genus Respirovirus , was detected in wild rodents from Thailand ( Fig. 2e ), confirming this virus not to be restricted to laboratory animals. No viruses belonging to this genus were detected in bats, but bat sera were found to react with respirovirus antigens ( Fig. 4b ), supporting previous assumptions that bats should carry closely related viruses [18] . Natural history of infection To compare organ-specific compartments of PV replication, virus concentrations in internal organs were determined in 22 African E. helvum bats infected with henipaviruses. The spleens of 21 of 22 animals tested positive with high virus concentrations, whereas all other internal organs as well as blood yielded virus at lower rates and concentrations ( Fig. 4d ). Organ distribution of morbilli-related PV in 28 rodents was strikingly different from that in bats, with broader and less organ-specific distribution of virus. Highest viral loads and most frequent virus detections in rodents were seen in the kidneys, and in bats in the spleens ( Supplementary Fig. S5 , Supplementary Tables S3 and S4 ). We next looked for evidence of continuous virus excretion on population level in bats [7] . A colony of Myotis myotis in Germany known to carry members of the Morbillivirus -related clade was monitored over 3 years for shedding of virus. Shedding rates and concentrations were constant over three observation periods throughout 2008 to 2010 ( Fig. 6 ). This colony was a maternity colony, and parturition times fell in the middle of observation periods but did not influence excretion, suggesting natural infection with little differences in shedding between young and adult animals. It was noted that this pattern was very different from that of measles virus in humans [19] , [20] . 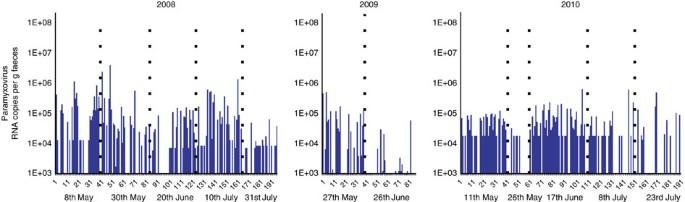Figure 6: Paramyxovirus (PV) faecal shedding over three reproductive seasons. PV faecal shedding over three reproductive seasons from 2008 to 2010 in aMyotis myotisbat maternity colony. Samples were obtained approximately every 3 weeks during the reproductive season from aMyotis myotismaternity roost located in the attic of a private house in Rhineland-Palatinate, Germany, throughout three sampling years (2008 to 2010). Sampling dates are shown onxaxes. Each sample was tested by specific real-time RT–PCR for morbilli-related PV. RNA concentrations per gram of faeces are given on theyaxis. Numbers on thexaxis represent individual faecal pools tested, consisting of five single faecal pellets each. Gaps between columns represent pools testing negative. Figure 6: Paramyxovirus (PV) faecal shedding over three reproductive seasons. PV faecal shedding over three reproductive seasons from 2008 to 2010 in a Myotis myotis bat maternity colony. Samples were obtained approximately every 3 weeks during the reproductive season from a Myotis myotis maternity roost located in the attic of a private house in Rhineland-Palatinate, Germany, throughout three sampling years (2008 to 2010). Sampling dates are shown on x axes. Each sample was tested by specific real-time RT–PCR for morbilli-related PV. RNA concentrations per gram of faeces are given on the y axis. Numbers on the x axis represent individual faecal pools tested, consisting of five single faecal pellets each. Gaps between columns represent pools testing negative. Full size image Interestingly, the morbilli-related viruses from M. myotis in Germany were also observed in genetically distant Coleura afra bats in Ghana. For several other PV clades, evidence of their association with bats beyond the limits of communicating social groups was obtained, as summarised in Fig. 7a and b . One pneumovirus, six henipaviruses and eight rubulaviruses were detected throughout several sampling years and sites across four different Western and Central African countries. Notably, widespread and constant detection of several viruses was observed in cave-roosting Rousettus aegyptiacus that do not participate in annual migrations and whose populations are isolated from each other ( Fig. 7c ). 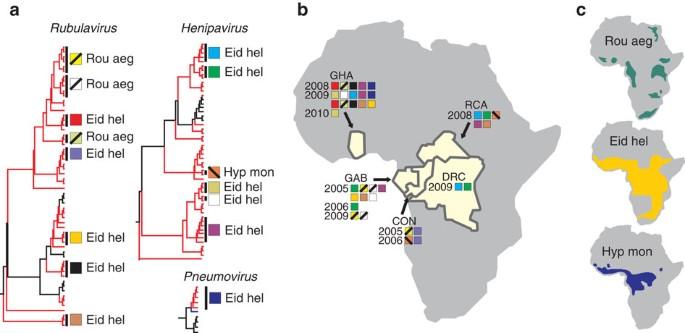Figure 7: Temporal and geographically linked PV detection in African fruit bat species. (a) Bat rubulaviruses, henipaviruses and pneumoviruses detected in more than one sampling site or year inRousettus aegyptiacus(Rou aeg),Eidolon helvum(Eid hel) andHypsignathus monstrosus(Hyp mon) are represented by different colours and symbols. (b) Detection of virus lineages in different sites and years. GHA=Ghana, CON=Republic of the Congo, DRC=Democratic Republic of Congo, RCA=Central African Republic. (c) Distribution of bat hosts as indicated by the IUCN red list (Bendaet al., 2008.Rousettus aegyptiacus.Mickleburghet al., 2008.Eidolon helvum. Mickleburghet al., 2008.Hypsignathus monstrosus. In: IUCN 2011. IUCN Red List of Threatened Species. Version 2011.2. (www.iucnredlist.org). Downloaded on 23 November 2011). Figure 7: Temporal and geographically linked PV detection in African fruit bat species. ( a ) Bat rubulaviruses, henipaviruses and pneumoviruses detected in more than one sampling site or year in Rousettus aegyptiacus (Rou aeg), Eidolon helvum (Eid hel) and Hypsignathus monstrosus (Hyp mon) are represented by different colours and symbols. ( b ) Detection of virus lineages in different sites and years. GHA=Ghana, CON=Republic of the Congo, DRC=Democratic Republic of Congo, RCA=Central African Republic. ( c ) Distribution of bat hosts as indicated by the IUCN red list (Benda et al ., 2008. Rousettus aegyptiacus. Mickleburgh et al ., 2008. Eidolon helvum . Mickleburgh et al ., 2008. Hypsignathus monstrosus . In: IUCN 2011. IUCN Red List of Threatened Species. Version 2011.2. ( www.iucnredlist.org ). Downloaded on 23 November 2011). Full size image To identify signs of PV-dependent disease in bats, paramount serum chemistry parameters were compared between infected and non-infected bats. No infection-dependent alterations were seen in concentrations of lactate dehydrogenase, gamma glutamyltransferase, aspartate aminotransferase, alanine transferase, bilirubin and albumin ( Supplementary Table S5 ). In summary, bats show an overwhelming PV diversity, continuous PV shedding without evidence of efficient immune control, signs of organ-specific replication and absence of PV-related pathogenicity. It was noted that these traits taken together are typical of viral ARs. Tracing hosts in PV phylogeny To extract information on hosts during the more recent evolution of extant mammalian PV, the most parsimonious hypothesis of historical host trait changes was reconstructed along the PV tree. To take topological uncertainty into account, this analysis was done on a large set of phylogenetic trees extracted from the terminal phase of an optimised Bayesian inference of phylogeny. The numbers of deduced transitions between ordinal categories of hosts including bats, rodents, primates, carnivores, ungulates and birds were estimated and averaged over >10,000 trees. To achieve a proper representation of PV from hosts other than bats and rodents, reference sequences were selected from GenBank so as to provide a maximal genetic diversity per ordinal host category ( Fig. 8a ). In summary, these analyses determined host switches from bats into other host categories to have occurred more often than switches originating from any other of these host categories ( Fig. 8b ). 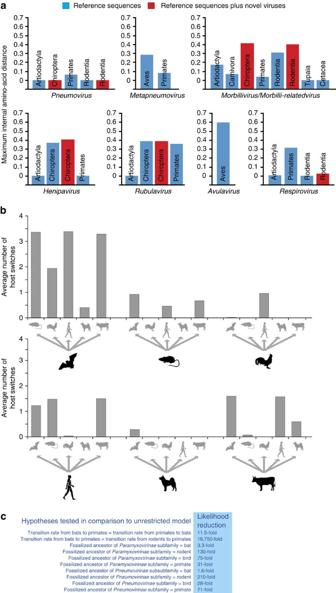Figure 8: Ancestral state reconstruction. (a) Patristic distances within PV genera detected per ordinal host categories (amino acid-based). Blue and orange colours represent diversification before and after inclusion of novel viruses from this study. (b) Summary of average host switches over ca. 10,000 trees as modelled by parsimony ancestral state reconstruction in Mesquite. Symbols on thexaxis depict donor (large symbols) and recipient hosts in the level of ordinal mammalian categories (bats, rodents, primates, carnivores, cetartiodactyls) and birds. Before the analysis, the rabies virus outgroup was removed, because this lyssavirus would have to be mapped to a bat host, biasing host state reconstruction for the root of the PV tree toward bats. Four single PV were removed because they were the only available PV in their particular host species (salmon, snake, dolphin, tupaia). (c) Summary of results from hypothesis testing using maximum likelihood (ML) ancestral state reconstruction in Bayestraits34. After analysis of 1,000 ML bootstrap trees, the trait change model was restricted by one of the ten criteria listed, and the resulting average likelihood of the restricted model was compared with that of the unrestricted model. The list shows the factor (n-fold) by which each restricted model was less likely than the unrestricted model (averaged over 1,000 bootstrap replicates of the underlying ML tree). Figure 8: Ancestral state reconstruction. ( a ) Patristic distances within PV genera detected per ordinal host categories (amino acid-based). Blue and orange colours represent diversification before and after inclusion of novel viruses from this study. ( b ) Summary of average host switches over ca. 10,000 trees as modelled by parsimony ancestral state reconstruction in Mesquite. Symbols on the x axis depict donor (large symbols) and recipient hosts in the level of ordinal mammalian categories (bats, rodents, primates, carnivores, cetartiodactyls) and birds. Before the analysis, the rabies virus outgroup was removed, because this lyssavirus would have to be mapped to a bat host, biasing host state reconstruction for the root of the PV tree toward bats. Four single PV were removed because they were the only available PV in their particular host species (salmon, snake, dolphin, tupaia). ( c ) Summary of results from hypothesis testing using maximum likelihood (ML) ancestral state reconstruction in Bayestraits [34] . After analysis of 1,000 ML bootstrap trees, the trait change model was restricted by one of the ten criteria listed, and the resulting average likelihood of the restricted model was compared with that of the unrestricted model. The list shows the factor (n-fold) by which each restricted model was less likely than the unrestricted model (averaged over 1,000 bootstrap replicates of the underlying ML tree). Full size image To achieve a statistical exclusion of alternative hypotheses regarding the host switching process, maximum likelihood analyses of ancestral state reconstruction were done under different model restrictions as summarised in Fig. 8c . All of these analyses suggested that bats but not rodents, primates or birds should be preferred donors of PV along the tree. Moreover, although assumptions of fossilised bat hosts at the root points of both PV subfamilies did not significantly reduce the model likelihood, all other fossilised host assumptions did. In this study, we have gathered evidence of bats being in close evolutionary and ecological relationship with several genera of mammalian PVs. The investigation of viral host associations can be a lengthy and controversial process that depends on targeted and ecologically informed sampling [21] , [22] , [23] , [24] , [25] , [26] , [27] , [28] , [29] . We believe that we have assembled the largest and most diversified single-sample set for investigating viruses in mammalian hosts. We focused on bats and rodents because of their unique properties among the mammals in terms of large social group sizes, intense social interaction and high population densities. Further criteria included high spatial mobility in the case of bats, and high population turnover in the case of rodents [1] , [2] , [4] , [30] . However, our data were not limited to these taxa, as an essential part of our analysis involved database-derived PV from a large range of other mammals as well as birds. The evolutionary distance between the analysed host taxa considerably exceeded that of either the bats or the rodents studied. It should be mentioned that PV entries in GenBank with and without our new data were not over-emphasising chiropteran or rodent hosts. As shown in Supplementary Fig. S6 , the majority of PV entries were from primates, birds, carnivores and ungulates. Even after addition of our novel data to GenBank data sets, the number of PV sequences from bats was just even with that from ungulates. Like almost all PVs currently contained in GenBank, our novel viruses were identified by RT–PCR and sequencing. PCR primers have an inherent bias due to their sequence specificity. We have applied a large range of published and own primer sets to compensate for this bias. Some of these have been thoroughly validated on clinical panels from a large range of hosts, confirming high sensitivity over a large genetic range of viruses [31] . More recent studies have suggested to improve the detection of novel viruses by hypothesis-free approaches such as random cDNA amplification from serum followed by deep sequencing [32] . Inclusion of such an approach in our study indeed revealed novel viral sequences that should be investigated further, but did not yield any PV. Low serum concentrations of PV RNA may have prevented detection, reminding us that hypothesis-free virus testing may not be sufficiently sensitive to enable comprehensive detection of viral flora [32] , [33] . ICTV currently lists 36 accepted PV species. Gene databases comprise more viruses, many of which are only partially sequenced and not classified into defined species ( Supplementary Tables S6 and S7 ). Although 83 clearly distinct PV taxa could be discriminated in our data set based on phylogeny, a classification criterion using a distance threshold comparable to that between HeV and NiV (7.0–7.5% in the L -gene fragment used) identified 66 independent novel taxonomic entities on the rank of tentative species to be represented in our data. Nevertheless, the number of novel taxa added to the PV phylogeny is unlikely to cause a bias toward bat- and rodent viruses in subsequent analyses of host associations. This is foremostly because reference sequences in these analyses were selected to maximise the patristic distance within each genus of PV ( Fig. 8a ). The algorithm underlying the parsimony-based ancestral state reconstruction only counts host switches once per resolved phylogenetic root point, irrespective of the number of depending leaves carrying identical traits. In general, probabilistic approaches such as ML- and Bayesian methods are considered more powerful than parsimony models for the reconstruction of character states evolving along phylogenetic branches [34] . However, this is mainly because probabilistic models take branch lengths into account, whereas parsimony-based methods only consider tree topology [34] . For the particular task of reconstructing viral host associations, we favour parsimony approaches out of theoretical considerations. First, we had to assume that host transition happens rarely and is unlikely to take place in a bidirectional manner, because of the fitness valley effect that will prevent host changes to be reversed easily [4] , [10] . In particular, viruses conquering a new host will leave behind population immunity in their original AR, preventing re-introduction, and making back and forward transitions (as well as host switching as a whole) a rare process [4] , [10] . Another argument was the uncertainty of deeper branch lengths in viral phylogenies [35] . More recent studies on non-retroviral RNA viruses invading mammalian germlines demonstrated tremendous discrepancies between apparent evolutionary rates of extant RNA viruses versus those of phylogenetic stem lineages [36] , [37] , [38] , [39] . Rate differences in deep branches will have great influence on probabilistic models, but will not affect parsimony assumptions. Even though recent findings of viral germline fossils comply with the idea that ancient PV may have existed in mammals [36] , [37] , [38] , [39] , such data are so far unavailable for PV, and we have not attempted in our analysis to determine the evolutionary origins of PV. Such an analysis would require a different approach to sampling, as viruses from taxa other than mammals and birds are currently underrepresented in databases. To attenuate the contribution of deep phylogenetic nodes, we have limited our analysis to an estimation of trait switches along trees, rather than inferring host associations for deep phylogenetic nodes. With this limitation in mind, we can conclude that bats have most often been the donors of those viruses currently encountered in other mammals. In spite of our preference for parsimony-based analysis, we have challenged this result by repetition in a probabilistic approach, testing the influence of alternative hypotheses by either restricting the trait change model or imposing fossilised ancestral state assumptions [40] . These analyses confirmed the results of the parsimony model and formally excluded other host hypotheses within the available data set. However, it should be mentioned that ancestral state analyses have not been systematically applied to the theoretical problem of viral host switching before. Many open questions remain, including the essential issue of developing significance criteria in host hypothesis testing. Only if complex data sets like ours become available for several other virus taxa, it will be possible to approach this major theoretical task. The current limitation, however, is in the sparse and incomplete biological sampling of habitat. Beyond phylogenetic analysis, we have identified traits of the natural history of infection that suggest a specific connection between PV and bats. The epidemiology of a morbilli-related virus was fundamentally different from that of measles virus in humans, or that of Rinderpest in cattle. Human measles is the prototype of viruses depending on steady transmission in sufficiently large social groups, potentially absent from isolated and remote populations [41] . Black [41] has defined this pattern of pathogen prevalence as the 'introduced disease' pattern, based on observations in isolated human tribes. Strikingly, in bats, the morbilli-related virus was excreted by adult animals at similar rates as by young animals, which is very untypical of morbilliviruses in other mammals. This pattern of prevalence was classified by Black [41] as 'endemic—high incidence, low morbidity', as exemplified in humans by hepatitis B virus or herpes viruses. Some researchers have argued that bats in general might deal with viral infections differently than other mammals [42] . However, we have recently described a variance of viral persistence patterns in bats that is congruent with observations in other mammals, with a typical 'introduced disease' pattern for astro- and coronaviruses, although a bat adenovirus in the same group of animals showed Black's 'endemic' pattern [41] , [43] . Adenoviruses provide a good template to explain the shedding pattern of the morbilli-related virus found in the present study, as they are known to persist in tissue and to be shed without signs beyond the acute phase of disease—a property determining the ability of viruses to persist in small populations [41] , [44] . Accordingly, the morbilli-related virus in our study was detected in a species of bats forming small- to medium-sized social groups ( M. myotis ), possibly requiring long-term excretion for virus maintenance on group level. This is rather untypical for morbilliviruses in other mammals that depend heavily on efficient transmission and sufficient group size to be maintained [30] , [41] , [45] . In this light, the difference in organ association between bats and rodents was quite interesting. Although PVs in rodents were associated with the kidney, favouring excretion, their highest concentrations and prevalences in bats were seen in the spleen. Although we have no further direct proof, this matches the concept that bat-borne PV might not as much depend on highly efficient transmission, but might routinely employ mechanisms of persistence to follow Black's 'endemic' pattern of prevalence [41] . This anomality might indeed identify bats as AR of these viruses. Moreover, the morbilli-related bat virus was detected in Europe, but also in an unrelated species forming rather small social groups in sub-Saharan Africa. Even though we have not been able to conduct longitudinal investigations of excretion in other PV genera, detection in groups without social connection as well as re-detection in subsequent years was seen also for rubula- and henipaviruses in this study. Detection of these viruses was not associated with changes in serum chemistry parameters, suggesting symptomless infection despite virus replication in internal organs, which may be regarded as typical for a virus in its natural host context that is not dependent on efficient horizontal transmission [4] , [7] , [46] . Beyond virus evolution and ecology, these data might have important implications for public health. HeV and NiV may be of African descent and have highly diversified relatives in Africa. These viruses might be associated with unrecognised disease, given the tremendous number of unresolved cases of encephalitis often ascribed to malaria in Africa [47] . Observed patterns of viral loads suggest that virus could be acquired during slaughtering of bats for alimentary purposes [48] , but possibly also through contact with ubiquitous bat faeces ( Supplementary Tables S3 and S8 ). It is for this same reason that the significance of Henipavirus -related agents in widely distributed bats in America deserves urgent further investigation. Moreover, the finding of agents serologically related to eradicable viruses, such as mumps, distemper and measles virus, is highly relevant in assessing perspectives and consequences of virus eradication [19] , [49] , [50] , [51] . Clearly, the bats investigated in this study carried viruses that were only similar but not identical to those agents endemic in humans or livestock. These new data therefore emphasise the importance of investigating possible transmission chains, as exemplified by the case of severe acute respiratory syndrome, in which an agent derived from bats was probably passed to humans by intermediate hosts such as carnivores [52] . In the case of the mumps-related bat virus, a direct antigenetic relatedness between human and bat viruses has been confirmed, and the close genetic proximity between both viruses suggests that even cross-neutralisation might be possible. In light of the still narrow representation of genetic diversity of bats covered in this study (ca. 7.5% of bat species), further research might reveal further bat-borne PV in close relationship to known pathogens of humans and livestock. If antigenic overlap exists, this could become relevant for virus eradication concepts. Relevant antigenic overlap would be defined by proof of cross-neutralisation between reservoir-borne and human or livestock pathogens. In this latter case, elimination of circulating virus and the subsequent cessation of vaccination might leave humans or livestock susceptible for reservoir-borne, antigenetically related viruses. Although these data identify a potential reservoir of important mammalian viruses, we can only begin to understand their true significance by functional investigation. Knowledge on the genetic range of pathogens carried by speciose small mammals may enable early recognition of zoonotic epidemics and rapid decision-making in the public health sector [53] , [54] . However, much more (and different) work needs to be done to actually assess and ameliorate zoonotic risks. The most relevant provision in this field is that epidemic risks emanating from wildlife virus reservoirs should trigger wildlife conservation rather than interference with wild animal populations [2] . Sampling and specimen preparation For all capturing, sampling and exportation of small mammal specimens, permission was obtained from the respective countries' authorities. Bats and rodents were identified by trained field biologists. Fresh bat droppings were collected on plastic film below roost sites [12] . Additionally, bats were caught with mist nets at roost or foraging sites, kept separately in bags until individual examination. Sampling relied on faecal pellets produced in bags, vein puncture for serum samples and mouth swabs. For organ samples, bats were euthanised with ketamine and dissected immediately. Rodents were caught with live traps or snap traps, euthanised and dissected. For faecal specimens, ca. 100 mg of faeces was suspended in 500 μl of RNAlater solution (Qiagen, Hilden, Germany) immediately after collection. Suspensions were homogenised by vortexing, and 50 μl were suspended into 560 μl of buffer AVL from the Qiagen Viral RNA Mini kit (Qiagen) and processed further according to the instructions of the manufacturer. For blood or serum samples, up to 140 μl (depending on the available quantity) were extracted. For solid organs, approximately 30 mg of tissue were homogenised in a TissueLyser (Qiagen) or a ball-mill tissue grinder (Genogrinder 2000, Spex Centripep), followed by extraction of RNA using the RNeasy Kit (Qiagen) or the ABI PRISM 6100 Nucleic Acid PrepStation (Applied Biosystems, Foster City, CA, USA). Elution volumes were generally 50 μl for serum/blood and faecal specimens, and 100 μl for tissue specimens. RNA specimens were subjected to molecular screening for PVs using a panel of oligonucleotides and RT–PCR assays listed in Supplementary Tables S9 and S10 . General conditions for RT–PCR About 100,000 RT–PCR reactions were done for this study, using ca. 100 different protocols. The basic formulation for 25-μl RT–PCR reactions used the Invitrogen SuperscriptIII OneStep RT–PCR kit (Invitrogen, Karlsruhe, Germany), with 800 nmol l −1 each of the respective first-round primers, 2.0 mmol l −1 MgSO 4 , 200 μmol l −1 deoxynucleoside triphosphates each, 1 μl enzyme mix, 1 μg bovine serum albumin, 10 U RNAseOut (Invitrogen) and 5 μl RNA extract. Amplification generally involved 30 min at 50 °C; 3 min at 95 °C; a touchdown element of 10 cycles of 15 s at 94 °C, 20 s starting at 64 °C with a decrease of 1 °C per cycle, and 40 s at 72 °C; and 35 cycles of 15 s at 94 °C, 20 s at 50 °C, and 40 s at 72 °C, with a final elongation step of 2 min at 72 °C. A volume of 50 μl second-round PCR reactions used 1 μl of first-round PCR product, with 1×Platinum Taq buffer (Invitrogen), 200 μmol l −1 deoxynucleoside triphosphates each, 2.0 mmol l −1 MgCl 2 , 800 nmol l −1 each of the respective second-round primers and 1 U Platinum Taq polymerase. All primers are listed in Supplementary Tables S9 and S10 . Virus quantification was done as described previously [55] . Briefly, amplicons from initial nested RT–PCR screening assays were TA-cloned (Invitrogen), plasmids purified and re-amplified with vector-specific oligonucleotides, and finally in vitro transcribed using the T7 promotor-based Megascript kit (Applied Biosystems, Darmstadt, Germany). Further details are available upon request from the authors. Next-generation sequencing Products of random cDNA amplification were loaded on 1.2% agarose gels. Primer dimers and large fragments (>700 bp) were removed, and amplicons were extracted from agarose gels. Fragments were end-repaired and a 454 sequencing library was constructed according to the GS Junior Rapid Library Preparation protocol (Roche, Penzberg, Germany). Emulsion PCR and sequencing reaction were performed as recommended by the manufacturer. Primer sequences were trimmed from each read, and all reads were aligned against the NCBI virus database using the tblastx local alignment algorithm in Geneious. All hits were scored and alignments with lengths less than 50 amino acids and a bit-score less than 40 were excluded. Serological assays Reactivity of human mumps virus with sera from different insectivorous and frugivorous bats was tested using mumps virus (strain Jones)-infected cells (Euroimmun EU38, Lubeck, Germany). Prototype PVs used for comparison included measles virus (strain Edmonston), RSV (RSV B Wash/18537/'62 (CH 18537)), parainfluenza virus 1 (PIV1, strain Sendai CPJ-3 13) and PIV2 (EU 18/9, strain Greer). Bat sera were diluted 1/40 and detection was done using first a goat anti-bat immunoglobulin (Ig) (Bethyl Laboratories, Montgomery, TX, USA) followed by a donkey anti-goat Ig conjugated to cyanine 3 (Dianova, Hamburg, Germany). Nuclei were stained with 4′,6-diamidino-2-phenylindole. Pictures were taken with a Motic fluorescence microscope (Zeiss). NiV indirect immunofluorescence was performed with NiV-infected Vero cells and a strain isolated from human brain tissue (kindly provided to AM by Jane Cardosa, Malaysia). Bat serum was diluted 1/10 and 1/40, and detection was done with the goat anti-bat Ig (Bethyl Laboratories) used for mumps immunofluorescence, followed by an Alexa Fluor 568 donkey anti-goat IgG (Invitrogen, Karlsruhe, Germany). A guinea pig anti-NiV serum was used as a positive control, followed by an Alexa Fluor 568 goat anti-guinea pig IgG. Serum chemistry A total of 119 native sera from E. helvum bats were analysed on a Dimension Vista automated analyzer (Siemens, Munich, Germany). The number of analysed parameters was limited by the amount of available sample material and included lactate dehydrogenase, alanine transferase, aspartate aminotransferase, gamma glutamyltransferase, albumin and total bilirubin. Phylogenetic analyses Nucleic acid alignments based on amino acid code were done in Mega4 ( www.megasoftware.net ). Gap-free coding nucleotide sequence alignments were generated containing the novel viruses as well as reference strains, using the complete deletion option in which any site containing gaps was deleted from the data set (see Supplementary Table S3 for a list of all reference strains with isolation years, host and GenBank accession number). The data set used for inference of Paramyxovviridae phylogenies comprised 559 nucleotide (nt). An additional analysis was done for only those rubulaviruses for which only a shorter 217 nt fragment could be amplified (see Fig. 2a , note that Supplementary Fig. S1 includes only rubulaviruses with complete 559 nt coverage). Bayesian phylogenies were calculated with MrBayes V3.2 [56] using amino acid sequences (WAG+G model) and nucleotide sequences (GTR+I+G model). Both analyses yielded identical topologies ( Fig. 2 and Supplementary Fig. S1 ). Convergence of chains was confirmed by the PSRF statistic in MrBayes [57] , as well as by visual inspection of individual traces using TRACER from the BEAST package [58] . Outgroups were Rabies virus (GenBank, NC_001542) for phylogenies, including the complete family Paramyxoviridae , Newcastle Disease virus for phylogenies of the genus Rubulavirus (GenBank, NC_002617) and Human Parainfluenzavirus 1 (GenBank, NC_003461) for the genera Henipa - and Morbillivirus . In parallel to the Bayesian analyses, maximum likelihood algorithms (WAG+G substitution model, 5 gamma categories and 1,000 bootstrap replicates) were applied using PhyML V3.0 [59] . Trees were visualised with FigTree V1.3.1 from the BEAST package [58] . Estimation of known PV taxa and their GenBank representation The known diversity of PVs and their hosts is shown in Supplementary Tables S6 and S7 . Supplementary Fig. S6 summarises the numbers of GenBank entries of PV by ordinal host groups. Threshold amino acid distance values for classifying phylogenetic branches were estimated by comparing the maximum amino acid distances within and between established PV species in the corresponding sequence fragments. Measles virus, mumps virus and RSV were selected to determine the maximum within-species distances per fragment, based on their good coverage in sequence databases. Maximum amino acid diversity within all publicly available mumps virus sequences was 1.6% in the translated 559 nt fragment, 5.4% for measles virus and 6.1% for RSV. For comparison, the amino acid divergence between the species HeV and NiV ranged from 7.0 to 7.5% in this fragment. Only taxa exceeding 7.0% amino acid distance were therefore counted as separate viruses. Ancestral state reconstruction Bayesian phylogenies were calculated using new PV sequences from this study, as well as a set of reference sequences from ordinal mammalian host categories (bats, rodents, primates, carnivores, ungulates), as well as birds. Reference sequences were selected from GenBank to maximise the genetic distance per ordinal host category ( Fig. 8 ). A total of 10,294 trees were extracted from the Bayesian phylogenetic analysis and ordinal mammalian host categories were assigned as noncontinuous state characters in Mesquite. Numbers of reconstructed trait changes according to an unordered parsimony assumption were summarised and averaged for each ordinal category over all trees. Reconstructed character traits at root points were also summarised and recorded. Hypothesis testing was done in Bayestraits [40] . This analysis was based on the ML phylogenetic tree shown in Supplementary Fig. S1 , including its 1,000 bootstrapped replicas. ML-based reconstructions of trait changes were calculated for each of the 1,000 replicas in Bayestraits, and the resulting median and mean values were listed in Excel. For hypothesis testing, the whole analysis was repeated under different restrictions that either synchronised the substitution rate assumptions of two different trait change processes, or that assumed defined common ancestor nodes within the tree to be fossilised to particular hosts. For each analysis, the median and mean log likelihoods were recorded. Relative model likelihoods of alternative hypotheses were compared by subtracting the respective median log likelihoods and linearising them. Accession codes: All virus sequences reported in this study have been deposited in the GenBank nucleotide database under accession numbers FJ971940 to FJ971960 , HQ660085 to HQ660195 and JF828295 to JF828309 . How to cite this article: Drexler, J.F. et al . Bats host major mammalian paramyxoviruses. Nat. Commun. 3:796 doi: 10.1038/ncomms1796 (2012).